Rb1 family mutation is sufficient for sarcoma initiation It is thought that genomic instability precipitated by Rb1 pathway loss rapidly triggers additional cancer gene mutations, accounting for rapid tumour onset following Rb1 mutation. However, recent whole-genome sequencing of retinoblastomas demonstrated little genomic instability, but instead suggested rapid epigenetic activation of cancer genes. These results raise the possibility that loss of the Rb1 pathway, which is a hallmark of cancers, might be sufficient for cancer initiation. Yet, mutation of the Rb1 family or inactivation of the Rb1 pathway in primary cells has proven insufficient for tumour initiation. Here we demonstrate that traditional nude mouse assays impose an artificial anoikis and proliferation barrier that prevents Rb1 family mutant fibroblasts from initiating tumours. By circumventing this barrier, we show that primary fibroblasts with only an Rb1 family mutation efficiently form sarcomas in nude mice, and a Ras-ZEB1-Akt pathway then causes transition of these tumours to an invasive phenotype. Although adult cancers are linked to a series of mutations that are thought to be acquired over a protracted period, pediatric tumours such as retinoblastoma frequently occur in a narrow developmental window and involve a limited number of mutations. Indeed, mutation of the second Rb1 allele is closely linked to onset of retinoblastoma, initially leading to a two-hit hypothesis where mutation of both Rb1 alleles was thought to be sufficient for retinoblastoma [1] . Although consistent additional mutations have yet to be identified in retinoblastoma, mutation of the Rb1 pathway has been linked to genomic instability, and it is thought that such instability precipitated by the Rb1 pathway loss triggers additional cancer gene mutations [2] . The rapid appearance of these mutations as a result of genomic instability is then thought to be responsible for the close linkage between mutation of the second Rb1 allele and onset of retinoblastoma. However, recent whole-genome sequencing of retinoblastomas demonstrated remarkably little genomic instability, and instead suggested that Rb1 mutation leads to rapid epigenetic derepression of cancer genes [3] . Along these lines, the Rb1 family, consisting of Rb1, p107 and p130, interacts with chromatin-modifying enzymes to repress transcription [4] . Such results raise the interesting possibility that loss of the Rb1 pathway, which is a hallmark of cancers, might be the only mutation required for cancer initiation. However, even though mutation of the Rb1 family in primary cells such as mouse embryonic fibroblasts (MEFs) leads to unrestricted proliferation, such mutation or inactivation of the Rb1 pathway has never been shown to be sufficient for tumour formation in xenograft experiments [5] , [6] . Instead, tumour initiation from Rb1 family mutant MEFs requires mutant Ras [6] . In solid tumours, unrestricted proliferation leads to loss of normal cell–extracellular matrix contacts, which can trigger anchorage-dependent cell death (anoikis) [7] . Anoikis is thought to be a hurdle for tumour initiation, and anchorage-independent survival (resistance to anoikis) in suspension culture or in soft agar is closely linked to the Ras pathway and the ability of mutant cells to form tumours in nude mice. Growth factor signalling through Ras is blocked when cells lose matrix contact [8] . Such signalling activates phosphoinositide-3 kinase (PI3K) and in turn Akt [9] , [10] , which blocks cell death by phosphorylating and inactivating proapoptotic factors such as Foxo3a, whose translocation to the nucleus is sufficient to initiate anoikis [11] . Formation of cell–cell contacts can substitute for loss of normal cell–matrix contacts to restore growth factor signalling, and such cell–cell contacts in the context of a primary tumour are thought to afford cancer cell resistance to anoikis, but this protection is lost as cells abandon the primary tumour to invade surrounding tissues [8] , [9] , [12] . Here we examined the effects of mutant Ras and cell–cell contacts on anoikis and tumour formation with Rb1 family mutant MEFs. We find that if cell–cell contacts are maintained, cells are protected from anoikis and the Rb1 family mutation is sufficient for tumour initiation in nude mice. However, cells that abandon the primary tumour die, preventing invasion. Mutant Ras allows for the survival of cells that abandon the primary tumour, thereby facilitating tumour invasion. Ras or cell–cell contacts block anoikis and cause Akt-S473 We found that the Rb1 family mutant MEFs (triple knockout (TKO) MEFs) showed initial resistance to anoikis when they were trypsinized to single cells and placed in suspension culture, but they failed to proliferate and lost viability after 2 days in suspension ( Fig. 1a,b ). By contrast, expression of mutant Ras in the TKO MEFs (Ras-TKO MEFs) led to proliferation and long-term survival in suspension ( Fig. 1a,b ), consistent with the tumorigenic phenotype of Ras-TKO MEFs in nude mice [6] . As cell–cell contacts restore growth factor signalling and resistance to anoikis to fibroblasts in suspension [8] , [12] , we asked whether such cell–cell contacts might block anoikis of TKO MEFs in suspension. We found that if TKO MEFs were pipetted or non-enzymatically dissociated (NED) to single cells, as opposed to trypsinization, the cells rapidly established cell–cell contacts in suspension ( Fig. 1a ). Moreover, similar to Ras-TKO MEFs where growth factor signalling is short circuited by mutant Ras, NED TKO cells that established cell–cell contacts were resistant to anoikis ( Fig. 1a ). Cells that failed to establish such contacts did not proliferate ( Fig. 1b ). Consistent with the importance of growth factor signalling for viability of TKO MEFs, removal of serum from the culture media led to a rapid loss of viability of NED cells in suspension, but it did not cause loss of viability of trypsinized single Ras-TKO MEFs, where the growth factor signalling pathway is short circuited ( Fig. 1a ). These results demonstrate that cell–cell contacts bypass a requirement for Ras mutation for proliferation and resistance to anoikis in suspension, but NED TKO MEFs that establish such cell–cell contacts are still dependent on serum growth factor signalling for proliferation and viability in suspension. 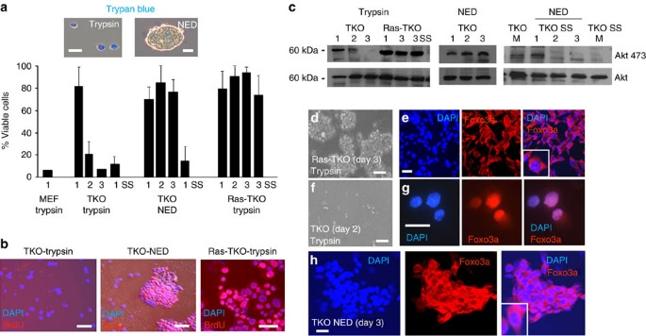Figure 1: Mutant Ras or cell–cell contacts prevent anoikis and cause constitutive Akt-S473 and cytoplasmic retention of Foxo3a in suspension culture. (a) Cells were placed in suspension culture and viability was assessed by trypan blue exclusion. Numbers indicate days in suspension culture. ‘NED’ indicates that single cells were generated non-enzymatically instead of by trypsinization, and these cells quickly formed cell–cell contacts in suspension. Trypan blue+single cells and trypan blue−associated cells are shown. ‘SS’ indicates cells in the absence of serum. DAPI, 4',6-diamidino-2-phenylindole. (b) Cells at day 2 in suspension culture were treated for 4 h with bromodeoxyuridine (BrdU) and then immunostained as described32. Note that TKO MEFs that failed to form cell–cell contacts did not incorporate BrdU. (c) Western blottings showing expression of total Akt and Akt-S473. ‘M’ indicates monolayer culture. (d) Phase image of Ras-TKO cells in suspension. (e) Immunostaining showing cytoplasmic retention of Foxo3a in Ras-TKO MEFs indafter 3 days in suspension. (f) Phase image of trypsinized TKO MEFs after two days in suspension. (g) Immunostaining showing translocation of Foxo3a to the nucleus in cells fromf. (h) Immunostaining showing cytoplasmic retention of Foxo3A in TKO MEFs with cell–cell contacts after 3 days in suspension. Scale bars, 20 μM. Error bars represent s.d. of three replicates. All results are representative of at least three independent experiments. Figure 1: Mutant Ras or cell–cell contacts prevent anoikis and cause constitutive Akt-S473 and cytoplasmic retention of Foxo3a in suspension culture. ( a ) Cells were placed in suspension culture and viability was assessed by trypan blue exclusion. Numbers indicate days in suspension culture. ‘NED’ indicates that single cells were generated non-enzymatically instead of by trypsinization, and these cells quickly formed cell–cell contacts in suspension. Trypan blue + single cells and trypan blue − associated cells are shown. ‘SS’ indicates cells in the absence of serum. DAPI, 4',6-diamidino-2-phenylindole. ( b ) Cells at day 2 in suspension culture were treated for 4 h with bromodeoxyuridine (BrdU) and then immunostained as described [32] . Note that TKO MEFs that failed to form cell–cell contacts did not incorporate BrdU. ( c ) Western blottings showing expression of total Akt and Akt-S473. ‘M’ indicates monolayer culture. ( d ) Phase image of Ras-TKO cells in suspension. ( e ) Immunostaining showing cytoplasmic retention of Foxo3a in Ras-TKO MEFs in d after 3 days in suspension. ( f ) Phase image of trypsinized TKO MEFs after two days in suspension. ( g ) Immunostaining showing translocation of Foxo3a to the nucleus in cells from f . ( h ) Immunostaining showing cytoplasmic retention of Foxo3A in TKO MEFs with cell–cell contacts after 3 days in suspension. Scale bars, 20 μM. Error bars represent s.d. of three replicates. All results are representative of at least three independent experiments. Full size image Akt can be activated by phosphorylation of S473 (Akt-S473) and T308 (Akt-T308), and these phosphorylated Akt forms have distinct functions [11] , [13] . Akt-S473 can inhibit anoikis by phosphorylation and inactivation of proapoptotic factors such as Foxo3a, whose nuclear translocation is sufficient to initiate anoikis [11] . We found previously that Akt-S473 accumulates in TKO MEFs with mutation of the Rb1 family, and that Akt-S473 levels are further increased in Ras-TKO MEFs [14] . Akt-S473 levels diminished as TKO MEFs lost viability in suspension, but Akt-S473 was maintained in Ras-TKO MEFs in suspension ( Fig. 1c ). Accordingly, Foxo3a was retained in the cytoplasm of Ras-TKO MEFs in suspension ( Fig. 1d,e ), whereas it accumulated in the nucleus of TKO MEFs in suspension ( Fig. 1f,g ). As with Ras-TKO MEFs, Akt-S473 was maintained in NED TKO MEFs that established cell–cell contacts in suspension and Foxo3a remained cytoplasmic ( Fig. 1h ), but Akt-S473 rapidly diminished when serum growth factors were removed ( Fig. 1c ). These results link resistance to anoikis to retention of Akt-S473 and cytoplasmic Foxo3a in suspension, and they demonstrate that serum growth factors are required for resistance of NED TKO MEFs to anoikis. Growth factor signalling or Ras maintains ZEB1 expression In carcinomas, induction of the transcription factor ZEB1 causes epithelial-to-mesenchymal transition (EMT) that triggers a migratory fibroblastic phenotype linked to invasion [15] . However, ZEB1 expression has also been linked to resistance to apoptosis, and lung and pancreatic cancer cells with a Ras mutation somehow become addicted to their elevated level of ZEB1 (refs 16 , 17 ). ZEB1 is repressed by the Rb1 family, and thus it is induced in TKO MEFs [18] . We found that ZEB1 expression diminished in TKO MEFs in suspension, but the expression was maintained and even increased in NED TKO MEFs that maintained cell–cell contacts in suspension ( Fig. 2a,b ). However, as with viability, ZEB1 expression diminished when serum growth factors were removed from NED TKO MEFs ( Fig. 2a,b ). By contrast, ZEB1 expression was not diminished when Ras-TKO MEFs were placed in suspension, nor did it diminish when serum growth factors were removed ( Fig. 2a,b ). Next, we examined the expression of ZEB1 in monolayer culture. ZEB1 expression was dependent on serum in both wild-type and TKO MEFs, but not in Ras-TKO MEFs ( Fig. 3a ). Together, these results demonstrate that although ZEB1 is derepressed in TKO MEFs with loss of the Rb1 family, its expression is still dependent on serum growth factors. 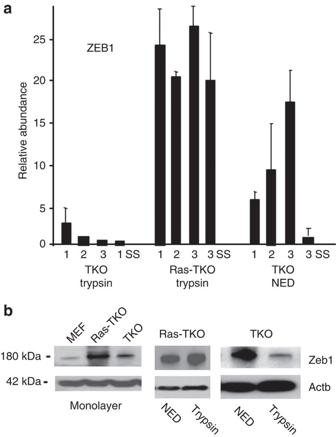Figure 2: Retention of ZEB1 expression in TKO MEF in suspension requires either cell–cell contacts and serum growth factor signalling, or mutant Ras. (a) Real-time PCR. Numbers indicate days in suspension and ‘SS’ indicates serum-starved cells as inFig. 1. (b) Western blottings showing the level of ZEB1. NED and trypsinized cells were in suspension for 2 days. The TKO MEF blot is exposed longer so that the level of ZEB1 in trypsinized cells can be seen (note the level of Actb). Error bars represent s.d. of three replicates. All results are representative of at least three independent experiments. Figure 2: Retention of ZEB1 expression in TKO MEF in suspension requires either cell–cell contacts and serum growth factor signalling, or mutant Ras. ( a ) Real-time PCR. Numbers indicate days in suspension and ‘SS’ indicates serum-starved cells as in Fig. 1 . ( b ) Western blottings showing the level of ZEB1. NED and trypsinized cells were in suspension for 2 days. The TKO MEF blot is exposed longer so that the level of ZEB1 in trypsinized cells can be seen (note the level of Actb). Error bars represent s.d. of three replicates. All results are representative of at least three independent experiments. 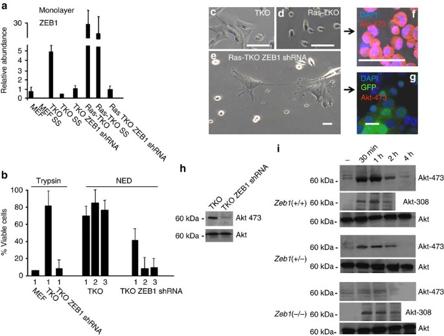Figure 3: ZEB1 is required for serum growth factor-induced Akt-S473 in wild-type MEFs and it mediates constitutive Akt-S473 in TKO and Ras-TKO MEFs. (a) Real-time PCR showing that ZEB1 expression is induced in TKO compared with wild-type MEFs, and that it is further induced in Ras-TKO MEFs. ZEB1 expression diminished in wild-type and TKO MEFs serum starved (SS) overnight, but serum starvation had no effect in Ras-TKO MEFs. Lentiviral knockdown of ZEB1 in TKO and Ras-TKO MEFs to a level similar to that in wild-type MEFs is shown. (b) Knockdown of ZEB1 restores anoikis in NED TKO MEFs. Numbers indicate days in suspension. (c–e) Phase images showing that knockdown of ZEB1 in Ras-TKO MEFs to a level similar to that in wild-type MEFs caused rapid loss of viability. Following shRNA lentiviral infections, most cells died and those that remained became large and flat (resembling senescent cells), and failed to proliferate. (f,g) Immunostaining of cells indandefor Akt-S473. Green fluorescent protein is expressed from the lentiviral shRNA vector. (h) Knockdown of ZEB1 in TKO MEFs leads to loss of constitutive Akt-S473. A western blotting showing total Akt and Akt-S473. (i) Wild-type orZEB1mutant MEFs35were serum starved overnight and then retreated with 20% serum for the indicated time. Western blottings showing total Akt, Akt-S473 and Akt-308. Error bars represent s.d. of three replicates. Scale bars, 20 μM. All results are representative of at least three independent experiments. Full size image Figure 3: ZEB1 is required for serum growth factor-induced Akt-S473 in wild-type MEFs and it mediates constitutive Akt-S473 in TKO and Ras-TKO MEFs. ( a ) Real-time PCR showing that ZEB1 expression is induced in TKO compared with wild-type MEFs, and that it is further induced in Ras-TKO MEFs. ZEB1 expression diminished in wild-type and TKO MEFs serum starved (SS) overnight, but serum starvation had no effect in Ras-TKO MEFs. Lentiviral knockdown of ZEB1 in TKO and Ras-TKO MEFs to a level similar to that in wild-type MEFs is shown. ( b ) Knockdown of ZEB1 restores anoikis in NED TKO MEFs. Numbers indicate days in suspension. ( c – e ) Phase images showing that knockdown of ZEB1 in Ras-TKO MEFs to a level similar to that in wild-type MEFs caused rapid loss of viability. Following shRNA lentiviral infections, most cells died and those that remained became large and flat (resembling senescent cells), and failed to proliferate. ( f , g ) Immunostaining of cells in d and e for Akt-S473. Green fluorescent protein is expressed from the lentiviral shRNA vector. ( h ) Knockdown of ZEB1 in TKO MEFs leads to loss of constitutive Akt-S473. A western blotting showing total Akt and Akt-S473. ( i ) Wild-type or ZEB1 mutant MEFs [35] were serum starved overnight and then retreated with 20% serum for the indicated time. Western blottings showing total Akt, Akt-S473 and Akt-308. Error bars represent s.d. of three replicates. Scale bars, 20 μM. All results are representative of at least three independent experiments. Full size image The link between integrins and growth factor receptors is well known [8] , [19] , [20] , [21] , [22] , [23] , [24] . Clustering of integrins on cell adhesion concentrates growth factor receptors to sites required for efficient signalling. Integrin ligation is required for integrin-associated focal adhesion kinase (FAK) activation in response to growth factors, and a lack of growth factor clustering and FAK activation in suspension causes a block in growth factor signalling. Such a loss of growth factor signalling in suspension then leads to loss of ZEB1 expression. By contrast, when mutant Ras is present, FAK and growth factor receptors are constitutively activated in an integrin-independent fashion, allowing for adhesion-independent growth factor signalling (and even growth factor-independent growth factor signalling). As growth factor signalling is short circuited with Ras mutation, Ras-TKO MEFs are not dependent on integrin ligation or growth factors for the maintenance of ZEB1 expression, providing for continued ZEB1 expression in suspension. Similar to adhesion to matrix, cell–cell contacts have also been shown to maintain growth factor signalling [12] , [23] , and this allows the maintenance of ZEB1 in NED TKO MEFs in suspension. But in contrast to Ras-TKO MEFs, NED TKO MEFs are still dependent on serum growth factors to maintain ZEB1. We then used lentiviral short hairpin RNA (shRNA) to knock down ZEB1 in TKO (TKO ZEB1 shRNA) and Ras-TKO (Ras-TKO ZEB1 shRNA) MEFs to a level similar to that in parent wild-type MEFs ( Fig. 3a ). TKO ZEB1 shRNA MEFs showed similar proliferation in monolayer culture but they lost viability more rapidly than TKO MEFs as single cells in suspension, and NED cells also underwent anoikis in suspension ( Fig. 3b ). Ras-TKO ZEB1 shRNA MEFs lost viability even in monolayer culture and could not be passaged ( Fig. 3c–e ). These results demonstrate that induction of ZEB1 seen in TKO MEFs is critical for resistance to anoikis, and that elevated ZEB1 is also critical for viability of Ras-TKO MEFs. ZEB1 is required for Akt-S473 phosphorylation We wondered whether induction of ZEB1 might be linked to constitutive Akt-S473 seen in TKO and Ras-TKO MEFs. Indeed, we found that constitutive Akt-S473 was lost with ZEB1 knockdown in both TKO and Ras-TKO MEFs ( Fig. 3f–h ). Although short-circuiting Ras mutations lead to constitutive activation of signalling pathways, including Erk and Akt, these pathways are normally induced only transiently by serum growth factors in wild-type cells [9] , [10] . Accordingly, when wild-type MEFs were serum starved and then retreated with serum growth factors, both Akt-S473 and Akt-T308 were induced within 30 min, and their level then diminished after 2 h ( Fig. 3i ). To determine whether ZEB1 might be important for this growth factor-induced phosphorylation of Akt in wild-type MEFs, we assessed the effect of ZEB1 mutation on this serum-induced Akt phosphorylation. Akt-S473 was diminished in a gene dosage-dependent manner in ZEB1 (+/−) and ZEB1 (−/−) MEFs, but Akt-T308 was unaffected by ZEB1 mutation ( Fig. 3i ). Surprisingly, these results demonstrate that a basal level of ZEB1 is necessary for serum growth factor-induced Akt-S473 in wild-type MEFs. However, induction of ZEB1 when the Rb1 pathway is lost and Ras is mutated somehow mediates constitutive Akt-S473. Because of this dependence of Akt-S473 on ZEB1, it is interesting to note that Akt can regulate the expression of the miR-200 family in a manner that depends on the balance between Akt1 and Akt2 (ref. 25 ). ZEB1 and miR-200 comprise a mutual repression loop [15] , raising the possibility that a balance of Akt isoform expression may also feedback to regulate the level of ZEB1. TKO and Ras-TKO MEFs are addicted to Akt Dependence of TKO and Ras-TKO MEFs on ZEB1, and in turn the requirement for ZEB1 for constitutive Akt-S473 in these cells, raised the possibility that elevated ZEB1 is important for viability, because these cells have become addicted to constitutively active Akt. To test this possibility, we used small interfering RNA to knock down the three Akt isoforms in wild-type, TKO and Ras-TKO MEFs. Knockdown of all three Akt isoforms led to rapid loss of Ras-TKO MEF viability in a monolayer culture ( Fig. 3a,b ). Moreover, loss of viability was also evident with knockdown of either Akt1 or Akt2, but the effect was most pronounced with loss of Akt1 ( Fig. 4a,b ). Likewise, knockdown of Akt in TKO MEFs also led to loss of viability. By contrast, knockdown of Akt isoforms in MEFs did not reduce viability in the monolayer culture ( Fig. 4a,b ). These results suggest that TKO and Ras-TKO MEFs have become addicted to constitutive Akt-S473, and the co-addiction to elevated ZEB1 reflects a requirement for elevated ZEB1 to somehow cause constitutive Akt-S473. 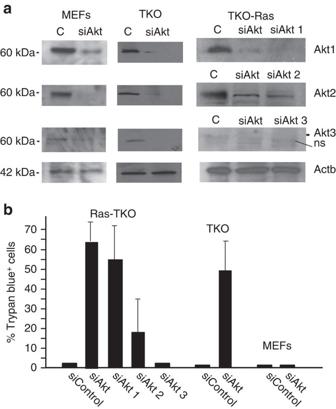Figure 4: TKO and Ras-TKO MEFs become addicted to Akt. (a) Western blottings showing the effects of small interfering RNA (siRNA) on the level of Akt isoforms. ‘C’ indicates a scrambled control siRNA. siAkt indicates a pan siRNA that targets all three isoforms. ‘ns’ indicates a nonspecific band. (b) Effect of Akt isoform knockdown on viability in monolayer culture. Cells were analysed 3 days after transfection for viability by trypan blue exclusion. Error bars represent s.d. of three replicates. All results are representative of at least three independent experiments. Figure 4: TKO and Ras-TKO MEFs become addicted to Akt. ( a ) Western blottings showing the effects of small interfering RNA (siRNA) on the level of Akt isoforms. ‘C’ indicates a scrambled control siRNA. siAkt indicates a pan siRNA that targets all three isoforms. ‘ns’ indicates a nonspecific band. ( b ) Effect of Akt isoform knockdown on viability in monolayer culture. Cells were analysed 3 days after transfection for viability by trypan blue exclusion. Error bars represent s.d. of three replicates. All results are representative of at least three independent experiments. Full size image However, how have TKO and Ras-TKO MEFs become addicted to Akt? Previously, we demonstrated that mutation of the Rb1 family in TKO MEFs led to elevated Akt-S473, but interestingly it also led to loss of Erk activation [14] . Moreover, introduction of Ras into these cells did not restore Erk activation. We provided evidence that constitutive Akt-S473 was feeding back to inhibit Raf, thus resulting in loss of Erk activation. We suggest that it is the switch from Erk signalling in wild-type MEFs to Akt signalling in TKO and Ras-TKO MEFs for proliferation/survival that is causing these cells to become dependent on Akt. ZEB1 regulates mTor expression to control Akt-S473 Akt-T308 is catalysed by Pdk1, but Akt-S473 is catalysed by mammalian target of rapamycin (mTor) in the context of mTor complex 2 (mTorc2) [11] , [13] . We found that mTor expression was low in MEFs, it was upregulated in TKO MEFs and further induced in Ras-TKO MEFs ( Fig. 5a ; ref. 14 ). Furthermore, mTor diminished along with Akt-S473 in TKO MEFs in suspension culture, and mTor expression was maintained along with Akt-S473 and resistance to anoikis in NED TKO MEFs and in Ras-TKO MEFs in suspension ( Figs 1b and 5a ). This induction of mTor then paralleled Akt-S473 and resistance to anoikis, raising the possibility that mTor expression might be rate limiting for the activity of mTorc2. We found that overexpression of mTor in MEFs (MEF-mTor) was sufficient for constitutive Akt-S473 and at least partial resistance to anoikis ( Fig. 5b,c ). Moreover, knockdown of mTor in TKO MEFs (TKO mTor shRNA MEFs) to a level similar to that in wild-type MEFs ( Fig. 5a,b ) diminished constitutive Akt-S473 and it restored anoikis within 24 h in suspension culture ( Fig. 5b,c ). These TKO mTor shRNA MEFs showed similar size and morphology to TKO MEFs, and their proliferation and viability in monolayer culture was also similar, implying that this level of mTor knockdown had not caused inactivation of mTorc1, which is critical for protein synthesis. However, mTor knockdown in Ras-TKO MEFs (also to a level similar to that in wild-type MEFs) led to a rapid loss of viability, as with knockdown of ZEB1 or Akt. Although overexpression of mTor led to constitutive Akt-S473 in MEF-mTor cells in monolayer culture, we found that removal of serum growth factors from the media still diminished Akt-S473 ( Fig. 5b ). Consistently, we also found that Akt-S473 was diminished in MEF-mTor cells in suspension culture where growth factor signalling is blocked ( Fig. 5b ). Taken together, our results demonstrate that induction of mTor is required to reach a threshold for constitutive Akt-S473, but mTorc2 is still dependent on serum growth factors or Ras mutation for PI3K-mediated activation. Interestingly, PI3K activation of mTorc2 involves association of mTorc2 with the ribosome, which might serve to link mTorc2 to cell metabolism [26] . As mTorc1 is involved in ribosome biogenesis, this finding may also serve to indirectly link mTorc2 activity to mTorc1. 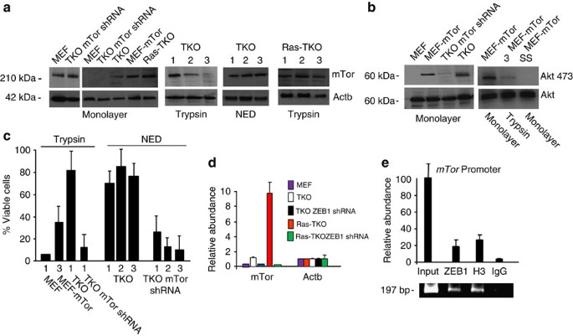Figure 5: ZEB1 regulates mTor expression to control Akt-S473. (a) Western blottings showing the expression of mTor. Numbers indicate days in suspension culture. The left-hand two lanes have five times more protein added so that the relative level of mTor can be compared in wild-type and TKO mTor shRNA MEFs. MEF-mTor indicates MEFs where mTor is overexpressed. (b) Western blottings showing that the level of mTor correlates with that of Akt-S473. However, Akt-S473 is still dependent on serum growth factors in MEF-mTor cells (SS), and it is lost when single trypsinized MEF-mTor cells are cultured in suspension for 3 days (3). (c) Knockdown of mTor in NED TKO MEFs to a level similar to that in wild-type MEFs restores anoikis. Viability is measured by trypan blue exclusion. Numbers indicate days in suspension. (d) Real-time PCR analysis showing that mTor mRNA is dependent on ZEB1. Similar to ZEB1, mTor is induced in TKO MEFs and it is further induced in Ras-TKO MEFs, and knockdown of ZEB1 diminishes mTor expression. (e) ChIP assay showing ZEB1 and histone H3 (positive control) binding to the mTor promoterin vivoin TKO MEFs. IgG indicates pre-immune rabbit antiserum as a control for ZEB1 antiserum. Input indicates total genomic DNA used for immunoprecipitation in the assays. Real-time PCR was used to quantify abundance, and a gel of PCR products is shown below. Error bars represent s.d. of three replicates. All results are representative of at least three independent experiments. Figure 5: ZEB1 regulates mTor expression to control Akt-S473. ( a ) Western blottings showing the expression of mTor. Numbers indicate days in suspension culture. The left-hand two lanes have five times more protein added so that the relative level of mTor can be compared in wild-type and TKO mTor shRNA MEFs. MEF-mTor indicates MEFs where mTor is overexpressed. ( b ) Western blottings showing that the level of mTor correlates with that of Akt-S473. However, Akt-S473 is still dependent on serum growth factors in MEF-mTor cells (SS), and it is lost when single trypsinized MEF-mTor cells are cultured in suspension for 3 days (3). ( c ) Knockdown of mTor in NED TKO MEFs to a level similar to that in wild-type MEFs restores anoikis. Viability is measured by trypan blue exclusion. Numbers indicate days in suspension. ( d ) Real-time PCR analysis showing that mTor mRNA is dependent on ZEB1. Similar to ZEB1, mTor is induced in TKO MEFs and it is further induced in Ras-TKO MEFs, and knockdown of ZEB1 diminishes mTor expression. ( e ) ChIP assay showing ZEB1 and histone H3 (positive control) binding to the mTor promoter in vivo in TKO MEFs. IgG indicates pre-immune rabbit antiserum as a control for ZEB1 antiserum. Input indicates total genomic DNA used for immunoprecipitation in the assays. Real-time PCR was used to quantify abundance, and a gel of PCR products is shown below. Error bars represent s.d. of three replicates. All results are representative of at least three independent experiments. Full size image Depending on promoter context, ZEB1 can bind the transcriptional co-activator p300 and serve as a transcriptional activator—p300 competes with the corepressor CtBP for binding to ZEB1, thereby eliminating default repression by ZEB1 (ref. 27 ). We found that mTor was induced along with ZEB1 in TKO and Ras-TKO MEFs ( Fig. 5d ), leading us to hypothesize that ZEB1 was responsible for induction of mTor. Indeed, knockdown of ZEB1 in TKO or Ras-TKO MEFs diminished mTor expression ( Fig. 5d ), demonstrating that mTor is positively regulated by ZEB1. Consistent with a direct effect of ZEB1 on mTor expression, we found multiple consensus E-box binding sites for ZEB1 in the mTor promoter, and ZEB1 bound to the mTor promoter in vivo in chromatin immunoprecipitation (ChIP) assays ( Fig. 5e ). We propose that ZEB1 is important for maintaining a threshold level of mTor in wild-type MEFs required for the generation of Akt-S473 in response to serum growth factors. Moreover, induction of mTor resulting from overexpression of ZEB1 in TKO and Ras-TKO MEFs leads to constitutive Akt-S473. TKO MEFs are able to maintain this constitutive Akt-S473 in suspension only if cells form cell–cell contacts to allow for growth factor signalling and induction of ZEB1. However, Ras-TKO MEFs are able to maintain constitutive Akt-S473 as single cells in suspension, because mutant Ras short circuits this growth factor signalling, thereby maintaining ZEB1 and thus mTor. Rb1 family mutation is sufficient for sarcoma initiation Next, we wondered how the effects on anoikis that we described above in suspension culture might relate to tumour formation. Beyond their role in carcinomas (for example, pancreatic and lung carcinomas), mutations in the Ras pathway are also important in progression of sarcoma [28] . When Ras-TKO MEFs were trypsinized to single cells and injected into nude mice, the cells were tumorigenic ( Table 1 ). Tumours were all histologically similar spindle-cell sarcomas and were highly invasive into the surrounding soft tissues ( Fig. 6 ). By contrast, TKO MEFs were not tumorigenic ( Table 1 ), demonstrating dependence on Ras for tumour initiation under these conditions. Table 1 Mutation of the Rb1 family in MEFs is sufficient for sarcoma initiation in nude mice and Ras mutation is required for invasion of these tumours. 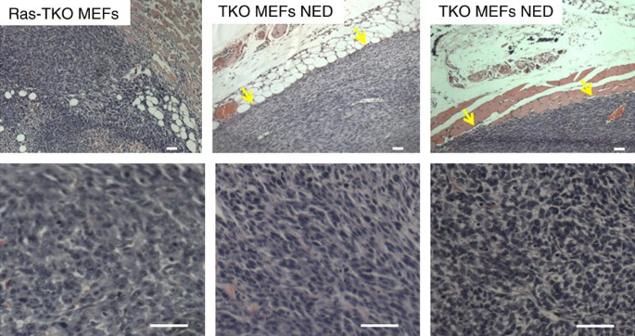Figure 6: Mutant Ras is required for invasion of NED TKO MEF sarcomas in nude mice. Tumour-host borders are shown above and higher power views of the tumour interior is shown below. Note the invasion of Ras-TKO MEF sarcomas into host skeletal muscle and adipose tissue, and the lack of corresponding invasion of NED TKO MEF sarcomas into the host tissues. Two different sections of NED TKO MEF tumours are shown to illustrate the lack in invasion into host skeletal muscle and adipose tissue. The border of NED TKO MEF tumours is shown by yellow arrows. Scale bars, 20 μM. Tumour histology is representative of results inTable 1. Full size table Figure 6: Mutant Ras is required for invasion of NED TKO MEF sarcomas in nude mice. Tumour-host borders are shown above and higher power views of the tumour interior is shown below. Note the invasion of Ras-TKO MEF sarcomas into host skeletal muscle and adipose tissue, and the lack of corresponding invasion of NED TKO MEF sarcomas into the host tissues. Two different sections of NED TKO MEF tumours are shown to illustrate the lack in invasion into host skeletal muscle and adipose tissue. The border of NED TKO MEF tumours is shown by yellow arrows. Scale bars, 20 μM. Tumour histology is representative of results in Table 1 . Full size image Mutation of Rb1 and p53 leads to sarcoma [29] , [30] . Although Rb1 mutant MEFs are arrested by p53, activation of p53 in TKO MEFs does not lead to growth arrest [5] , [6] , demonstrating that p53 function is dependent on the Rb1 family. Accordingly, mutation of Rb1 and p107 is sufficient for sarcoma in vivo [31] . Yet, TKO MEFs were not tumorigenic in nude mice ( Table 1 ). On the basis of our findings in suspension culture, we reasoned that trypsinization of TKO MEFs to single cell suspensions for injection into nude mice might block proliferation and induce anoikis, thereby preventing tumour initiation. Therefore, instead of trypsinization, NED TKO MEFs were injected into nude mice to allow the potential for cell–cell contacts to establish. Remarkably, NED TKO MEFs formed tumours, and the tumour size was similar to those formed with Ras-TKO MEFs ( Table 1 ). Furthermore, the tumours were all spindle-cell sarcomas similar to those formed by Ras-TKO MEFs ( Fig. 6 ). A similar injection of NED TKO ZEB1 shRNA MEFs did not lead to tumour formation ( Table 1 ), demonstrating that induction of ZEB1 in the TKO MEFs is required for tumour initiation. Likewise, NED TKO mTor shRNA MEFs did not form tumours ( Table 1 ). Taken together, our results provide evidence that Rb1 family mutation in MEFs is sufficient for sarcoma formation in nude mice when cell–cell contacts are maintained. Ras mutation is required for tumour invasion Although the tumours formed with Ras-TKO MEFs and NED TKO MEFs were similar in size and histology, Ras-TKO MEF tumours were highly invasive into the surrounding soft tissues, whereas those formed with NED TKO MEFs were all non-invasive ( Table 1 and Fig. 6 ). These results provide evidence that mutant Ras in the TKO MEFs is required for the tumour cells to transition to an invasive phenotype. Next, we immunostained TKO NED and Ras-TKO tumours for the proliferation marker Ki67 and Akt-S473. Both tumours showed Ki67 + and Akt-S473 + cells throughout the tumour, but there was a slightly higher overall proliferation rate in the Ras tumours ( Fig. 7a,b ). As TKO NED tumours were non-invasive, we wondered whether cells at the edge of the tumour might show diminished Ki67 and Akt-S473 as they detached from the tumour, causing cell death and thereby preventing invasion. As anticipated, we found that invading Ras-TKO cancer cells expressed both Akt-S473 and Ki67, but TKO NED tumours also expressed Akt-S473 and Ki67 at the tumour edge ( Fig. 7a ). One interpretation is that similar to that in suspension culture, cells that leave the tumour die rapidly and thus they are not detected. Nevertheless, the TKO tumours lack invading cells. 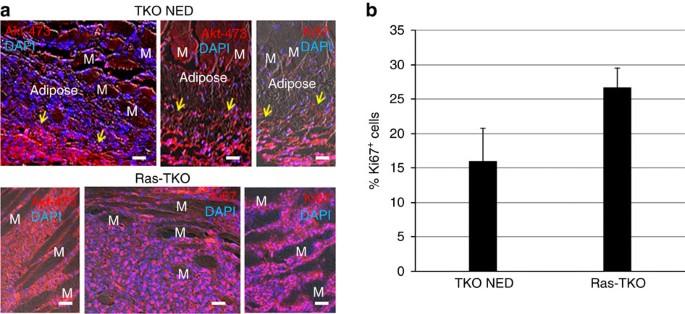Figure 7: Proliferation and Akt-S473 in TKO NED and Ras-TKO tumours. (a) Immunostaining for Ki67 and Akt-S473 in TKO NED and Ras-TKO tumours inFig. 6. Arrows indicate the tumour border and ‘M’ indicates host muscle tissue. (b) The percentage of Ki67+cells was counted in four different regions of three different tumours. Scale bars, 20 μM. Error bars represent s.d. of three replicates. Figure 7: Proliferation and Akt-S473 in TKO NED and Ras-TKO tumours. ( a ) Immunostaining for Ki67 and Akt-S473 in TKO NED and Ras-TKO tumours in Fig. 6 . Arrows indicate the tumour border and ‘M’ indicates host muscle tissue. ( b ) The percentage of Ki67 + cells was counted in four different regions of three different tumours. Scale bars, 20 μM. Error bars represent s.d. of three replicates. Full size image We propose that trypsinizing and suspending cells in suspension before injection places an artificial anoikis and proliferative barrier on tumorigenesi1s in nude mice by disrupting the potential for cell–cell contacts, which, we demonstrate, are critical for tumour initiation with some cells. Differences in sarcoma initiation and invasion in our experiments with TKO and Ras-TKO MEFs are mirrored by properties of the two cells in suspension culture ( Fig. 8a–c ). Although TKO MEFs survive when they form cell–cell contacts in suspension, which we put forth as analogous to a primary tumour, cells that do not form these contacts undergo rapid anoikis. We suggest that these non-associated cells are representative of potentially invasive cells that shed from the primary tumour. In the case of Ras-TKO MEFs, Ras induction of ZEB1, upregulation of mTor and resulting constitutive Akt-S473 allows these cells to survive and invade surrounding tissues. In contrast, dependence of TKO MEFs on cell–cell contacts within the primary tumour to maintain ZEB1, mTor and Akt-S473 leads to anoikis of cells when they are shed from the tumour, thereby blocking invasion. 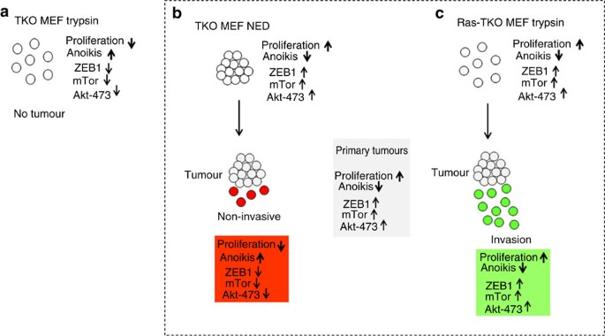Figure 8: Trypsinizing cells in suspension before injection into nude mice places an artificial proliferation and anoikis barrier on tumour initiation. (a) When TKO MEFs are trypsinized and placed in suspension, the single cells are no longer growth factor responsive, leading to downregulation of ZEB1 and, in turn, loss of Akt-S473. These cells stop proliferation and undergo anoikis, preventing them from forming tumours when injected into nude mice. (b) Maintaining cell–cell contacts in TKO MEFs in suspension (TKO MEF NED) allows growth factor signalling to maintain ZEB1 and thus constitutive Akt-S473, and the cells continue to proliferate and are resistant to anoikis. These cells form sarcomas when injected into nude mice, and as in suspension culture we propose that cell–cell contacts between TKO MEFs within the primary tumour allow growth factor signalling to maintain elevated ZEB1 and constitutive Akt-S473. However, as with single cells in suspension culture, TKO MEFs that abandon the primary tumour (red circles) lose growth factor signalling, leading to loss of ZEB1 and in turn Akt-S473. These cells then stop proliferation and undergo anoikis, preventing their invasion. (c) Mutant Ras short circuits growth factor signalling, leading to retention of ZEB1 and thus constitutive Akt-S473 when Ras-TKO MEFs are trypsinized and placed in suspension culture. These cells continue proliferation and are resistant to anoikis. They form tumours in tumour mice and, similar to that in suspension culture, cells that dissociate from the primary tumour (green circles) maintain ZEB1 and Akt-S473; thus, they continue proliferating and are resistant to anoikis, allowing them to invade surrounding tissues. These results place anoikis as a critical hurdle for transition to tumour invasion, as opposed to tumour initiation. We suggest that Ras mutation acts at this step of tumour invasion by blocking anoikis of cells that abandon the primary tumour. Moreover, this effect of Ras is mediated by its ability to maintain ZEB1 expression under these conditions, which in turn causes constitutive Akt-S473. Figure 8: Trypsinizing cells in suspension before injection into nude mice places an artificial proliferation and anoikis barrier on tumour initiation. ( a ) When TKO MEFs are trypsinized and placed in suspension, the single cells are no longer growth factor responsive, leading to downregulation of ZEB1 and, in turn, loss of Akt-S473. These cells stop proliferation and undergo anoikis, preventing them from forming tumours when injected into nude mice. ( b ) Maintaining cell–cell contacts in TKO MEFs in suspension (TKO MEF NED) allows growth factor signalling to maintain ZEB1 and thus constitutive Akt-S473, and the cells continue to proliferate and are resistant to anoikis. These cells form sarcomas when injected into nude mice, and as in suspension culture we propose that cell–cell contacts between TKO MEFs within the primary tumour allow growth factor signalling to maintain elevated ZEB1 and constitutive Akt-S473. However, as with single cells in suspension culture, TKO MEFs that abandon the primary tumour (red circles) lose growth factor signalling, leading to loss of ZEB1 and in turn Akt-S473. These cells then stop proliferation and undergo anoikis, preventing their invasion. ( c ) Mutant Ras short circuits growth factor signalling, leading to retention of ZEB1 and thus constitutive Akt-S473 when Ras-TKO MEFs are trypsinized and placed in suspension culture. These cells continue proliferation and are resistant to anoikis. They form tumours in tumour mice and, similar to that in suspension culture, cells that dissociate from the primary tumour (green circles) maintain ZEB1 and Akt-S473; thus, they continue proliferating and are resistant to anoikis, allowing them to invade surrounding tissues. These results place anoikis as a critical hurdle for transition to tumour invasion, as opposed to tumour initiation. We suggest that Ras mutation acts at this step of tumour invasion by blocking anoikis of cells that abandon the primary tumour. Moreover, this effect of Ras is mediated by its ability to maintain ZEB1 expression under these conditions, which in turn causes constitutive Akt-S473. Full size image There is controversy regarding the origin of cancer stem cells/cancer-initiating cells in tumours. However, we have demonstrated previously that cells with cancer stem cell properties can be induced from the population of cancer cells, and this induction required ZEB1 (ref. 32 ). Recently, Weinberg and colleagues [33] published similar findings, demonstrating that ZEB1 modulates a reversible transition of existing breast cancer cells to cancer stem cells. There is mounting evidence that early invasive/metastatic cells in pancreatic and breast cancer have induced ZEB1 and show properties of cancer stem cells [33] , [34] . Remarkably, in Ras-induced pancreatic cancer, invasive/metastatic ZEB1 + cells with cancer stem cell properties were already evident at the stage of precancerous prostatic intraepithelial neoplasia (PIN) lesion before a frank tumour had developed [34] . Together, these studies provide evidence that in at least some cancers, cancer stem cells can arise from the existing cancer cell population through induction of ZEB1, and they link these cancer stem cells to early invasion/metastasis. Cell culture Rb1 family mutant MEFs from four separate embryos were obtained from Sage et al . [6] and used with similar results. Cells were cultured in DMEM with 10% heat-inactivated fetal bovine serum [14] . Ras-TKO MEFs were created by infection with human H- ras V12 mutant retrovirus (a gift from Dr R Mitchell, University of Louisville, Louisville, KY, USA). Ras activity was assessed using the EZ-Detect Ras Activation Kit (Pierce Biotechnology, Rockford, IL) and glutathione S -transferase fusion protein containing the Ras-binding domain of Raf [14] . Tumour formation in nude mice Mouse studies have been approved by the University Institutional Animal Care and Use Committee. Cells were trypsinized, pipetted with a P200 pipetman, or treated with cell dissociation buffer obtained from Invitrogen (Carlsbad, CA), to generate single cells in suspension. Cells in suspension were injected subcutaneously into the hind limb of nude mice [31] . Tumours were fixed in 10% buffered formalin, embedded in paraffin and sectioned for haematoxylin and eosin staining or immunostaining. Real-time PCR and ChIP assays RNA was extracted using TRIzol (Invitrogen). Complementary DNA was synthesized using the Invitrogen RT Kit according to the manufacturer’s protocol. SYBR Green real-time quantitative PCR was performed using the Mx3000P Real-Time PCR System (Stratagene, Cedar Creek, TX) according to the manufacturer’s instructions. PCR primers are shown in Table 2 . Three independent samples, each in triplicate, were analysed for each real-time PCR condition, and products were analysed for size by agarose gel. ChIP assays were based on the Upstate Biotechnology protocol ( http://www.millipore.com/userguides/tech1/789mrn ) using formaldehyde to cross-link genomic DNA. Polyclonal antiserum for ZEB1 (ref. 35 ), histone H3 and histone H4 (Santa Cruz Biotechnology, Inc., Santa Cruz, CA) were used for immunoprecipitation. Equal amounts of anti-IgG or pre-immune serum were used as negative controls, whereas histone H4 served as a positive control. ChIP PCR reactions were similar to those described above for real-time PCR using primer sets ( Table 2 ) to amplify promoter sequences of mTor . Table 2 PCR primers used in this study. Full size table Gene knockdowns To generate a lentivirus expressing ZEB1 or mTOR shRNA [14] , [32] , a primer containing a Zeb1 shRNA sequence (5′-CTGTCTAGACAAAAAAAGACAACGTGAAAGACAATCTCTTGAATTGTCAAACACGTTGTC TTGGGGATCTGTGGTCTCATACA-3′) or an mTOR shRNA sequence (5′-CTGTCTAGACAAAAGAGATGGAGGAGATCACCCTCTCTTGAAGGGTGATCTCCTCCAT CTCGGGGATCTGTGGTCTCATACA-3′) was used with a T3 primer to amplify a 500-bp fragment containing the H1 promoter using the pSuper vector as a template. The resulting PCR product was digested with Spe I and Xba I, and cloned back into the lentiviral vector digested with Nhe I. We first cloned the shRNA sequence into a cytomegalovirus–green fluorescent protein lentiviral vector, where its expression was driven by the mouse U6 promoter [32] . Briefly, the shRNA construct was generated by synthesizing an 83-mer oligonucleotide containing the following: a 19-nucleotide sense strand and a 19-nucleotide antisense strand, separated by a nine-nucleotide loop (5′-TTCAAGAGA-3′); a stretch of five adenines as a template for the Pol III promoter termination signal; 21 nucleotides complementary to the 3′-end of the Pol III U6 promoter; and a 5′-end containing a unique Xba I restriction site. The long oligonucleotide was used, together with a sp6 oligonucleotide (5′-ATTTAGGTGACACTATAGAAT-3′), to PCR-amplify a fragment containing the entire U6 promoter plus shRNA sequences; the resultant product was digested with Xba I and Spe I ligated into the Nhe I of the lentivirus vector, and the insert was sequenced to ensure that no errors occurred during the PCR or cloning steps. Lentiviral particles were produced by a four-plasmid transfection system [32] . Briefly, 293T cells were transfected with the lentiviral vector and packaging plasmids, and the supernatants, containing recombinant pseudolentiviral particles, were collected from culture dishes on the second and third days after transfection. TKO MEFs and Ras-TKO MEFs were transduced with these lentiviral particles expressing shRNAs targeting ZEB1. A transduction efficiency of near 100% was achieved based on green fluorescent protein-positive cells. Beyond these original shRNAs, we used five additional shRNA lentiviruses with different shRNA sequences obtained from Open Biosystems, for knockdowns with similar effects. Lentivirus with a scrambled shRNA sequence 5′-CAACAAGATGAAGAGCACCAATCTCTTGAAT TGGTGCTCTTCATCTTGTTG-3′ was used as a control—this control sequence was blasted against all mouse RNA sequences to ensure that it did not target a messenger RNA. Mouse Akt isoform small interfering RNAs were from OriGene. Immunostaining Cells were washed with PBS, fixed with 4% formaldehyde for 10 min and then washed again with PBS. The cells were then treated with methanol at −20 °C for 10 min and blocked with 4% goat serum at room temperature for 1 h. Cells were incubated with primary antibody overnight at 4 °C. The following primary antibodies were used: rabbit anti-phospho-Akt (Ser 473) polyclonal antibody (1:10; Cell Signaling Technology, Inc.; Boston, MA), rabbit anti-Foxo3a polyclonal antibody (1:10; Santa Cruz Biotechnology, Inc.), rabbit anti-mTor polyclonal antibody (H-266) (1:10; Santa Cruz Biotechnology, Inc.) and rabbit anti-Ki67 polyclonal antibody (1:20; Novus Biologicals). The next day, cells were washed with PBS followed by incubation with secondary antibody (Alexa Fluor goat anti-rabbit IgG; Invitrogen) for 1 h at room temperature. Images were captured with a Zeiss confocal microscope. Western blotting Cell extracts were prepared by washing with cold PBS and adding 100 μl of lysis buffer (Pierce Biotechnology) with protease inhibitor cocktail (Sigma-Aldrich, Saint Louis, MO), followed by high-speed centrifugation. Protein concentration was assayed by the Bradford Method (Bio-Rad Laboratories, Richmond, CA). Forty micrograms of protein from each sample was subjected to electrophoresis on a 4–20% gradient SDS–polyacrylamide gel (Bio-Rad Laboratories) and transferred to nitrocellulose membrane (GE Healthcare Biosciences, Piscataway, NJ). Membranes were blocked for 1 h in 5% powdered milk and 0.1% Tween 20, and then incubated overnight with primary antibody, followed by a 1-h incubation with horseradish peroxidase-conjugated secondary antibody (Pierce Biotechnology), and detection was done with enhanced chemiluminescence (Perkin Elmer, Waltham, MA). The following antibodies were used: rabbit anti-phospho-Akt (Ser 473) polyclonal antibody (1:1,000; Cell Signaling Technology, Inc.), rabbit anti-phospho-Akt (Thr 308) polyclonal antibody (1:1,000; Santa Cruz Biotechnology, Inc.), rabbit anti-Akt polyclonal antibody (1:1,000; Santa Cruz Biotechnology, Inc.), rabbit anti-FRAP polyclonal antibody (1:1,000; Santa Cruz Biotechnology, Inc.), rabbit anti-phospho-Raf-1 (Ser 259) polyclonal antibody (1:1,000; Santa Cruz Biotechnology, Inc.) and anti-ZEB1 (1:1000; a gift from Douglas S Darling) [35] . How to cite this article: Liu, Y. et al . Rb1 family mutation is sufficient for sarcoma initiation. Nat. Commun. 4:2650 doi: 10.1038/ncomms3650 (2013).